A distinct ripple-formation regime on Mars revealed by the morphometrics of barchan dunes Sand mobilized by wind forms decimeter-scale impact ripples and decameter-scale or larger dunes on Earth and Mars. In addition to those two bedform scales, orbital and in situ images revealed a third distinct class of larger meter-scale ripples on Mars. Since their discovery, two main hypotheses have been proposed to explain the formation of large martian ripples—that they originate from the growth in wavelength and height of decimeter-scale ripples or that they arise from the same hydrodynamic instability as windblown dunes or subaqueous bedforms instead. Here we provide evidence that large martian ripples form from the same hydrodynamic instability as windblown dunes and subaqueous ripples. Using an artificial neural network, we characterize the morphometrics of over a million isolated barchan dunes on Mars and analyze how their size and shape vary across Mars’ surface. We find that the size of Mars’ smallest dunes decreases with increasing atmospheric density with a power-law exponent predicted by hydrodynamic theory, similarly to meter-size ripples, tightly bounding a forbidden range in bedform sizes. Our results provide key evidence for a unifying model for the formation of subaqueous and windblown bedforms on planetary surfaces, offering a new quantitative tool to decipher Mars’ atmospheric evolution. From decimeter-scale ripples to decameter-scale or larger dunes, aeolian (windblown) bedforms are ubiquitous across Mars’ desert landscapes. In addition to small-scale ripples, a distinctly larger class of meter-scale ripples was discovered on Mars from observations made by NASA’s Curiosity rover [1] , [2] (Fig. 1 ). On Earth, meter-scale ripples only form in the presence of wide or bimodal grain-size distributions, with two grain-size populations moving through two distinct transport modes—saltation and creep [3] . However, many large ripples on Mars lack a concentration of coarser grains that would be transported in creep near their crests [4] , [5] , [6] , [7] , [8] and thus cannot be explained by bimodal transport [3] . Fig. 1: Dunes and ripples on Mars. a Impact ripples superimposed on large wind ripples atop Namib dune, Gale Crater, Mars. (Curiosity rover Mastcam mosaic; credit: NASA/JPL-Caltech/MSSS/Thomas Appéré). b Large ripples superimpose barchan dunes, Hellespontus Montes, Mars (−41.4°N, 44.6°E; High Resolution Imaging Science Experiment (HiRISE) image PSP_007676_1385). c Detailed view of large ripples with wavelength ~2 m (orange rectangle in panel ( b )). Full size image Two models have been proposed to date to explain the co-existence of the two distinct ripple scales on Mars. Under the first model, large ripples would result from the continuous growth of small ripples from saltation-driven impact splash, enabled by low dynamic wind pressures on Mars (i.e., they would be impact ripples [9] ). However, ripples with intermediate sizes (~20–80 cm) were not observed to be active in relatively well sorted sand [1] , [2] , [5] , [6] , [10] , contradicting the model’s prediction that a continuum of ripple sizes should exist between those of small and large ripples. Furthermore, the crest-to-crest spacing (or wavelength, λ , Fig. 1 ) of large martian ripples was shown to decrease with increasing atmospheric density ( ρ f ), following a trend that is quantitatively consistent with predictions from a scaling relationship developed for subaqueous drag ripples [1] , [5] , [11] . Consistent with those observations, another model [12] suggests that large wind ripples form from the same hydrodynamic instability [13] as windblown dunes and subaqueous bedforms. Specifically, the scale separation between Mars’ windblown large ripples and dunes (and between subaqueous ripples and dunes) would arise from a hydrodynamic anomaly [14] , [15] that prevents the growth of bedforms with intermediate wavelengths [12] . Under hydrodynamically smooth flow conditions, a hydrodynamic anomaly (hereafter referred to as the Hanratty anomaly) was shown to arise as bedform size increases [14] , [15] . This anomaly is linked to the way pressure gradients are balanced within the inner boundary layer in response to bedform topography; it arises when the flow within the inner boundary layer (disturbed by bedform topography) remains laminar upstream of the bedform crest but becomes turbulent downstream as turbulent fluctuations amplify [12] . The anomaly thus depends on the turbulent response imparted by the bedform and takes place as the disturbed flow in the inner boundary layer transitions from fully laminar to fully turbulent across the bedform length, as has also been proposed for drag bedforms [11] . This transitional regime is defined by a range in bedform-scale Reynolds number, \({{{{{{\rm{Re}}}}}}}_{ \lambda }=\frac{ \lambda {u}_{*}}{\nu }\) (with \(\lambda\) the bedform wavelength, \({u}_{*}\) the wind shear velocity, and \(\nu\) the flow’s kinematic viscosity), which may vary with sediment transport conditions [11] , [12] . This hydrodynamic anomaly was reported from a single set of well controlled experiments where the bed, unlike natural dunes, was non-erodible [14] , [15] ; however, its existence has not yet been demonstrated in nature where bed topography arises from flow-driven sediment transport and deposition. Existing theory for the hydrodynamic instability that generates dunes is formulated for ideal transverse (i.e., migrating roughly perpendicularly to average crestline orientation) periodic dunes with unlimited sediment supply. Barchans dunes are transverse bedforms that form under relatively unimodal winds, but they occur under limited sediment supply [16] . However, the size of nascent barchan dunes, approximated here as the smallest dunes in their immediate environment (2nd percentile in bins of size 60 km 2 ), is expected to be similar to the wavelength of incipient periodic transverse dunes that would arise under the same flow conditions but greater sediment supply [17] . Thus, because they are prevalent across Mars [18] , [19] , [20] , [21] , [22] and are ideal objects for machine-learning assisted detection due to their unique isolated crescentic shape (Methods), they offer a unique opportunity to investigate the environmental controls on dune sizes and shapes (Fig. 1b ) across Mars’ surface as a test to bedform-formation theory [12] . Specifically, if Mars’ large ripples and dunes form from the same hydrodynamic instability, both the wavelength of large ripples (as was evidenced from orbital imagery [1] ) and the size of the smallest barchan dunes should decrease with increasing atmospheric density following a similar trend. In turn, the observed decrease in bedform wavelength should be characterized by a power-law exponent strictly greater than −1 ( \(\lambda \propto {\rho }_{f}^{-1}\) for barchans whose length, like on Earth, scales with transport saturation length [23] , [24] , [25] , the spatial scale over which sand flux equilibrates to its saturated value) and smaller or equal to −1/2 (i.e., bedform size is influenced by the viscous length scale, \(\frac{\nu }{{u}_{*}}\) ; \(\lambda \propto {\rho }_{f}^{-1/2}\) for sand transport at threshold conditions; Methods) [11] . In this work, we test this hypothesis by generating a global dataset of barchan morphometrics (Figs. S1 – S2 ) on Mars to reveal geospatial trends as they relate to the global near-surface atmospheric circulation and local environmental conditions. Our extensive dataset, which includes over a million barchan dunes previously outlined by an instance segmentation neural network and validated using a comprehensive manually processed dataset [26] (Fig. 2a and Figs. S3 – S5 ), reveals the size of barchan dunes on Mars decreases with increasing atmospheric density, similar to the wavelength of large ripples. Our results support the hypothesis [1] , [12] that large ripples on Mars form from the same hydrodynamic instability as dunes, indicating that ancient aeolian bedforms can be used to reconstruct the density of Mars’ atmosphere at the time of sediment deposition. Fig. 2: Morphometrics of barchan dunes on Mars. a Example of automatically detected barchans on Mars (−42.20°N, −31.89°E). Outlines (white) were identified by the neural network in Mars Reconnaissance Orbiter (MRO) Context Camera (CTX) [42] images. The red dashed outline shows a detection that was discarded by our algorithm on the basis of the absence of a convexity deffect. Red and green crosses indicate the automatically detected tails and horns, respectively. b – g Correlations between morphometric parameters on Mars (red) and Earth (blue). Line histograms indicate the marginal distribution of each parameter. Regression lines are shown as red (Mars) and blue (Earth) lines; R 2 values were computed as the square of Pearson’s correlation coefficient. Full size image Global morphometrics of barchan dunes on Mars We find that the relationships between dune width (W), length (L), height (H) and volume (V; Fig. 2b–g ) on Mars closely follow terrestrial scaling laws. Dune length and width display a near-linear relationship ( \(L\propto {W}^{1.011\pm 0.001}\) , \({R}^{2}=0.52\) , \(p \, < \, 0.01\) ). Our estimates of dune height, which are derived from imagery and are sensitive to illumination, show greater scatter but remain close to linear functions of planform dune dimensions. A stronger correlation between dune length and height hints that dune length is a more robust predictor of height than width, which shows greater scatter ( \(H\propto {L}^{0.858\pm0.001},\,{R}^{2}=0.52,\,{p} \, < \, 0.01{;\; H}\propto {W}^{0.702\pm0.004},\,{R}^{2}=0.29,\,{p} \, < \, 0.01\) ). Correlations between the planform dimensions of barchans and their estimated volumes show relatively low scatter. When fitted with a power law, dune volume follows a near-cubic relationship with both width and length ( \(V\propto {W}^{2.577\pm 0.001},{R}^{2}=0.72,\,{p} \, < \, 0.01\) and \(V\propto {L}^{2.669\pm 0.002},\,{R}^{2}=0.81,\,{p} \, < \, 0.01\) ). We find that barchan dunes on Mars and Earth follow similar linear relationships between length and width ( \(L\propto 0.9W\) ), height and length \((H\propto 0.11L)\) , and height and width ( \(H\propto 0.08W\) ) [27] , [28] , and follow cubic scaling laws of \(V\sim \frac{1}{37}{L}^{3}\) and \(V\sim \frac{1}{42}{W}^{3}\) , which are similar to barchan dunes on Earth [28] . These similarities between barchan scaling laws previously derived on Earth to those we derived using our comprehensive dataset on Mars demonstrates that dunes on Mars and Earth share important morphodynamics [29] and could be used to constrain general physical laws of aeolian transport on both planets. Furthermore, we find that the size of the smallest barchan dunes on Mars decreases with increasing atmospheric density over the density range investigated here (~0.01–0.03 kg/m 3 ; Fig. 3 ; Figs. S4 – S5 ). This trend can be described with power laws in terms of dune length, \(L\sim {{\rho }_{f}}^{-0.68\pm0.03}\) , and dune width, \(W\sim {{\rho }_{f}}^{-0.63\pm0.03}\) ( \({R}^{2}=0.34\) and \({R}^{2}=0.31\) , respectively; errors indicate a 95% confidence interval). The observed data scatter around these correlations are both a consequence of local environmental conditions and the automatic nature of the measurements. For example, dune width—a measurement more sensitive to illumination—displays greater scatter than dune length near the pole. A comparison of atmospheric densities obtained using the hypsometric equation (Equation M3; “Methods”) and from a global circulation model during seasons of active sand transport revealed that seasonal variations in atmospheric density do not have a significant impact on these results (Supplementary Information; Fig. S7 ). Fig. 3: Dune length (blue-to-yellow circles) and large-ripple wavelength (light purple [1] and dark green circles [36] ) decreases with increasing atmospheric density. Ripple data follows a previously derived scaling relationships for drag ripples [5] ; best-fit power law to an updated global compilation of dark-toned large-ripple wavelength has an exponent of −0.63 (green dashed line) [35] . The width of the hydrodynamic anomaly (gray shade) was calculated for a 125 μm grain size [7] and assuming that wind shear velocity is at the transport threshold [49] (Methods), using the model of ref. 12 . The statistical significance of the regression slope was computed using a Wald Test, and errorbars (narrower than line width) indicate a 95% confidence interval. Each dot in the figure represents the 2nd percentile dune length in equal-area bins (60 km 2 ). Full size image First surveys of barchan dunes on Mars, prior to the Mars Reconnaissance Orbiter [18] , [30] , were limited by image resolution and reported average dune sizes of ~500 m [18] , [30] . 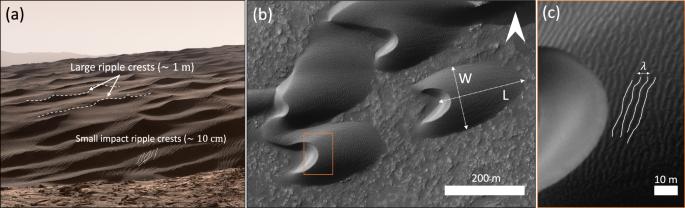Fig. 1: Dunes and ripples on Mars. aImpact ripples superimposed on large wind ripples atop Namib dune, Gale Crater, Mars. (Curiosity rover Mastcam mosaic; credit: NASA/JPL-Caltech/MSSS/Thomas Appéré).bLarge ripples superimpose barchan dunes, Hellespontus Montes, Mars (−41.4°N, 44.6°E; High Resolution Imaging Science Experiment (HiRISE) image PSP_007676_1385).cDetailed view of large ripples with wavelength ~2 m (orange rectangle in panel (b)). Here, we find that small barchan dunes dominate the dataset, and consequently report much smaller values of average dune sizes: \(220{{{{{\rm{m}}}}}}\) at mid ( \(70^\circ {{{{{\rm{S}}}}}}-70^\circ {{{{{\rm{N}}}}}}\) ) and \(160\) m at high (> \(70^\circ {{{{{\rm{N}}}}}}\) , Table 1 ) latitudes. The large number of small dunes at high northern latitude decreases the average dune size near the pole relative to lower-latitude dunes (70°S–70°N). The pixel size of the Context Camera (CTX) mosaic we employ (5–6 m/pixel) is much smaller than the typical size of dunes, precluding the possibility that dunes were not detected due to insufficient spatial resolution. Table 1 Summary of barchan morphometrics on Mars and comparison with Earth (rounded to nearest integer; P 2 and P 98 denote the 2nd and 98th percentiles, respectively) Full size table The size and shape of barchan dunes are controlled by a complex interplay between both the global properties of the atmosphere and local perturbations, e.g., from topography, dune-dune interactions, local variations in excess wind shear velocities, or near-surface volatiles [24] , [29] , [31] , [32] (Supplementary Information). Such perturbations lead to the observed scatter in dune dimension for any given atmospheric density, whereas the first-order control of atmospheric properties is reflected by the global relationship between dune dimensions and atmospheric density when local effects are averaged (Fig. 3 ). While the higher relative abundance of smaller dunes at high northern latitudes is likely due to the lower elevation, and thus, higher atmospheric pressure throughout Mars’ northern lowlands, the greater scatter in dune size in that region could potentially arise from cryogenic processes, which were found to affect the saltation saturation length scale and, as a result, dune growth (Fig. S9 ) [33] , [34] . Importantly, both the wavelength of large dark-toned ripples [35] , [36] and length of the smallest barchan dunes decrease with increasing atmospheric density, robustly and tightly bounding the wavelength gap that would arise from hydrodynamic theory (Fig. 3 ; Figs. S6 – S8 ). The best-fit power law between dune size and atmospheric density has an exponent close to −2/3—the same value as that empirically derived for subaqueous ripples [1] , [5] , [11] . In addition, the departure from a true inverse relationship, as would be expected if dune size was solely controlled by transport saturation length [1] , [5] , [11] , confirms that the viscous length scale \(\left(\frac{\nu }{{u}_{*}}\right)\) impacts the initial size of martian dunes as well, lending quantitative support to the hydrodynamic model of ref. 11 . Thus, these observations are readily consistent with a hydrodynamic origin of large martian ripples [1] , [5] , [6] , [12] , [37] . Under this hypothesis, the smallest bedforms arising from that hydrodynamic anomaly on Mars—meter-scale ripples—are about an order of magnitude smaller than terrestrial protodunes. Like larger aeolian dunes, these meter-scale ripples may grow through time, but their growth would be limited by the hydrodynamic anomaly arising from Mars’ low-density atmosphere (which increases the atmosphere’s kinematic viscosity, explaining their analogy to subaqueous ripples), triggering erosion at the crest of bedforms with wavelengths of a few meters to several decameters. Whereas their size is not the most favored on Mars (i.e., their growth rate is not highest), ~80 m-scale incipient dunes may also form (and subsequently grow) because the formation of smaller dunes that could prevent their inception is precluded by the hydrodynamic anomaly [12] . Specifically, the observed decrease in large-ripple and dune sizes with increasing atmospheric density is quantitatively consistent with the existence of a hydrodynamic anomaly defined by a constant range in bedform-scale Reynolds number, \({{{{{{\rm{Re}}}}}}}_{ \lambda }=\frac{ \lambda {u}_{*}}{\nu } \sim 5\times {10}^{3}-6\times {10}^{4}\) (where \({u}_{*}\) is the wind shear velocity; “Methods”) under martian surface conditions. This remarkable agreement between model predictions and observations on Mars’ surface strongly supports the hypothesis that large martian ripples are more analogous to drag ripples and aeolian dunes than to aeolian impact ripples [1] , [5] , [12] . Thus, ancient aeolian sandstones may disclose the density of Mars’ atmosphere at the time of sediment deposition through reconstructions of windblown bedform sizes [1] , [38] , offering prime exploration targets to unravel the evolution of Mars’ early atmosphere and surface environments. Detection of barchan dunes on Mars with machine learning Our global database of barchan dune morphometrics on Mars was compiled using a convolutional neural network (CNN), providing the fullest description of martian barchan dunes to date. Data were processed with minimal human intervention. Whereas manually processed data typically present higher accuracy per sample, the errors in the average morphometrics reported here and that were potentially introduced by our automatic analysis are mitigated in a central-limit theorem sense. In addition, the global coverage of our data provides an outlook into otherwise elusive spatial trends in dune morphology. Dune fields on Mars were globally cataloged and classified manually in prior studies [20] , [22] , and the morphology of individual barchan dunes was studied locally [18] , [29] . 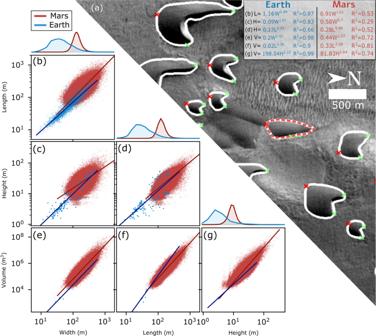Fig. 2: Morphometrics of barchan dunes on Mars. aExample of automatically detected barchans on Mars (−42.20°N, −31.89°E). Outlines (white) were identified by the neural network in Mars Reconnaissance Orbiter (MRO) Context Camera (CTX)42images. The red dashed outline shows a detection that was discarded by our algorithm on the basis of the absence of a convexity deffect. Red and green crosses indicate the automatically detected tails and horns, respectively.b–gCorrelations between morphometric parameters on Mars (red) and Earth (blue). Line histograms indicate the marginal distribution of each parameter. Regression lines are shown as red (Mars) and blue (Earth) lines;R2values were computed as the square of Pearson’s correlation coefficient. 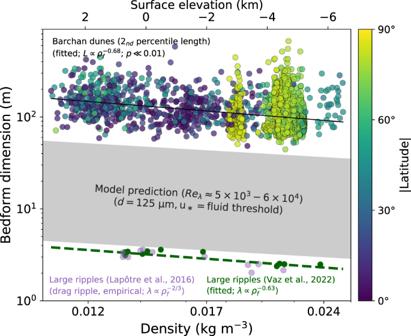Fig. 3: Dune length (blue-to-yellow circles) and large-ripple wavelength (light purple1and dark green circles36) decreases with increasing atmospheric density. Ripple data follows a previously derived scaling relationships for drag ripples5; best-fit power law to an updated global compilation of dark-toned large-ripple wavelength has an exponent of −0.63 (green dashed line)35. The width of the hydrodynamic anomaly (gray shade) was calculated for a 125 μm grain size7and assuming that wind shear velocity is at the transport threshold49(Methods), using the model of ref.12. The statistical significance of the regression slope was computed using a Wald Test, and errorbars (narrower than line width) indicate a 95% confidence interval. Each dot in the figure represents the 2nd percentile dune length in equal-area bins (60 km2). These studies did not generate datasets sufficient in size in which the smallest dunes could be identified in a statistically robust way. Such a survey of the smallest dunes on Mars requires an exhaustive sample of dunes. However, compiling such an extensive dataset has been challenging to date due to the large number of dunes on Mars and the time-consuming nature of manual measurements. Barchan dunes are ideal objects for machine-learning assisted detection because they appear as isolated units and their unique crescentic shape makes them more readily detectable by both humans and machines compared to other types of dunes [26] . Traditional computer vision techniques rely on sharp image gradients for object detection and are inaccurate when the objects and their environment have similar colors or textures [39] . Recently, deep machine learning algorithms have revolutionized object detection in images, achieving human-like abstraction [40] . These CNNs excel at supervised learning tasks such as finding a set of parameters that, given a set of inputs, best reproduces a set of expected outputs. To extract dune contours on Mars, we used Mask R-CNN, a state-of-the-art supervised instance segmentation CNN [41] . We first manually labeled isolated barchan dunes in a set of images extracted from the global MRO CTX (5–6 m/pixel [42] ) mosaic [43] . We elected to exclude connected barchanoidal ridges that are more difficult to analyze automatically. Using this dataset, we optimized the parameters of Mask R-CNN through training, until its accuracy (the mean average precision evaluated using a separate test dataset [26] ) reached 77%. Our dataset included 1074 images of barchan dunes, uniformly selected across the martian surface to obtain a well balanced dataset. The training and validation datasets were composed of 80 and 20% of the total manually labeled data, respectively. Mean average precision (mAP) was determined from an additional test dataset composed of 50 images. To avoid overfitting, we employed image augmentations (rotations, image saturation, contrast), as well as L2 regularization. The full set of hyperparameters of the trained model can be found in ref. 26 . While training the model further would have likely resulted in higher accuracy and better outlier detection, we found this mAP value sufficient for our goal of characterizing the first-order morphometrics of barchan dunes on Mars. The trained model was then used to detect isolated barchans in the global CTX mosaic [43] . A full discussion of training process and model evaluation is provided in ref. 26 , and a discussion of the errors associated with our statistical analysis is provided in the Supplementary Information. Extraction of dune morphometrics from dune outlines Of the 137,111 CTX images extracted automatically from the global CTX mosaic and examined by the CNN, 55,674 were found to contain at least one instance of an object identified as an isolated barchan dune. To measure the morphometrics of each identified dune, we automatically identified six reference points along the dune contour—the slipface center, the horns’ apexes, the tail, and the dune sides [28] (Fig. S1 ). The slipface center (middle of the base of the slipface) was identified as the deepest convexity defect along the dune contour. Horn apexes were mapped as the two intersection points between the dune contour and its convex hull closest to the slipface center. The tail of the dune was set as the point furthest away from the slipface along the dune’s stoss (Supplemental Material). Finally, the sides of the dunes were detected as the two extreme points along the dune contour in the direction perpendicular to a vector drawn between the tail and the slipface center (Fig. 1 and Fig. S1 ). The dune length was measured as the distance between the tail and the slipface center, the dune width as the distance between its sides, and the horn lengths (not discussed in this work) as the distances between the horn apexes and a line passing through the slipface center, normal to the tail-slipface vector. We estimated dune height by multiplying the horizontal length of the slipface (measured from the brink to the base of the slipface, in map view) by the tangent of 30° as a representative angle of repose for martian aeolian sand [6] , and dune volume, as the product of H /2 (as a proxy for the average height of all points along the dune’s surface) and basal area within the dune outline (Fig. S1 ). Data filtering To increase the robustness of our compilation, we filtered our dataset as follows: (1) Between 70°S–70°N, we only used images of areas previously mapped as dune fields [20] , [22] . This was done to save computation time – since our goal is not to detect new barchan dunes on Mars but to characterize the morphology of dunes on Mars on a global scale. (2) Because barchans tend to occur in fields rather than as solitary landforms, we discarded images containing less than three objects to remove potentially spurious detections. (3) Upon manually inspecting our results, we found that the model misclassified some dark sublimation-driven features at southern polar latitudes, such as Dalmatian spots and spiders [44] , as barchans. Consequently, we elected to discard dunes in latitudes poleward of 70°S. (4) By removing dunes with detection-confidence levels outputted by the detection algorithm lower than 70%, and dunes with convexity defects smaller than 2.5% of total dune length ( L + mean horn length). The latter step removed many isolated objects erroneously identified as dunes, but also isolated dome dunes, which are excluded from this study. Our choice of 70% confidence is based on trial and error and visual inspection of the detected objects. Upon filtering, our final dataset contained 646,134 dunes (covering an area of about \(15\times {10}^{3}\,{{{{{{\rm{km}}}}}}}^{2}\) ), roughly 97% of which are located poleward of 70°N. We use orthogonal distance regression [45] to describe various correlations between dune morphometrics as best-fit power laws (Fig. 2b–g ). To filter for intra-crater dunes south of 70°N, we used craters locations and diameters as mapped manually [46] . We find that south of 70°N, 3,819 dunes in our database are located in the inter-crater terrain, and 15,309 dunes are found within craters. Validation of automatically computed morphometrics The quality of our final dataset was validated manually by comparing automatically measured morphometrics to manually measured morphometrics in CTX images using JMARS [47] . Additionally, the extracted morphometrics data was validated with a smaller test dataset of manually measured barchan morphometrics on Mars [48] (Figs. S3 – S4 ) as well as with individual HiRISE digital terrain models (Supplementary Information; Fig. S5 ). Width of the hydrodynamic anomaly on Mars Under martian surface conditions, the gap in bedform sizes arising from the Hanratty anomaly was predicted to correspond to \({{{{{{\rm{Re}}}}}}}_{ \lambda } \sim 5\times {10}^{3}-6\times {10}^{4}\) 12 . We expressed the width of the hydrodynamic anomaly in terms of bedform wavelength, \(\lambda\) , as 
    λ=ν/u_∗Re_λ,
 (1) where \({{{{{{\rm{Re}}}}}}}_{ \lambda } \sim 5\times {10}^{3}-6\times {10}^{4}\) and wind shear velocity, \({u}_{*}\) , was estimated to a first order as the transport fluid threshold, \({u}_{*{{{{{\rm{f}}}}}}}\) , 
    u_∗f=√(ρ_s-ρ_f/ρ_fgdθ),
 (2) where \({\rho }_{s}\,\approx\, 2900\) kg/m 3 is the density of basaltic sediment grains, \(g\,\approx\, 3.71\) m/s 2 is the surface acceleration of gravity, \(d\,\approx\, 125\) μm is sediment grain diameter [7] and \(\theta=0.01\) is the critical Shields number as constrained from Mars-like low-pressure wind tunnel experiments [49] . We tested the sensitivity of the derived bedform-gap width to the chosen threshold model by comparing this formulation with additional fluid threshold models [16] , [50] , and found this choice does not affect our conclusions (Figs. S6 – S8 ). Because dune-forming winds ought to be larger than the impact threshold for sand transport ( \({u}_{*{{{{{\rm{i}}}}}}}\) ), we also calculated the width of the Hanratty gap by equating \({u}_{*}\) to values derived from impact-threshold models [25] , [51] , [52] (not shown) and found a similar overlap between predicted bedform gaps and the observed range of missing bedform wavelengths on Mars. We note that these results could be used to constrain formative wind shear velocities within a given dune field from the observed range of missing bedform wavelengths. Estimation of atmospheric density from topography We computed the surface atmospheric density, \({\rho }_{f}\) , on Mars assuming an isothermal ideal-gas CO 2 atmosphere ( \({m}_{{{{{{\rm{c}}}}}}{{{{{{\rm{o}}}}}}}_{2}}=44.01{{{{{\rm{g}}}}}}/{{{{{\rm{mol}}}}}}\) ) with surface pressure of \({P}_{0}=610{{{{{\rm{Pa}}}}}}\) , temperature \({T}_{0}=230{{{{{\rm{K}}}}}}\) and a scale height of H = 12 km [53] , 
    ρ_f=ρ_0exp (-z/H)
 (3) where \({\rho }_{0}=\left({P}_{0}{m}_{{{{{{{\rm{co}}}}}}}_{2}}\right)/\left(R{T}_{0}\right)\) , \(R=8.3145{{{{{\rm{J}}}}}}{{{{{{\rm{mol}}}}}}}^{-1}\,{{{{{\rm{K}}}}}}\) is the ideal gas constant, and the height, \(z\) , was measured using Mars Orbiter Laser Altimeter data. To produce Fig. 3 , we binned atmospheric density and dune sizes between latitudes - \(70^\circ {{{{{\rm{N}}}}}}\) and \(90^\circ {{{{{\rm{N}}}}}}\) in equal-area spatial bins of 60 km 2 (1° near the equator) and plotted the 2nd percentile of dunes length in the bin as a function of its atmospheric density calculated using the mean bin elevation. We confirmed that the statistical properties of the distributions do not vary significantly for bin sizes of 15–60 km 2 . Furthermore, we find that data from dunes located inside impact craters display a slightly higher scatter than dunes outside of craters, a likely results of crater topography on local wind conditions [54] , sediment accumulation, and other environmental factors (Supplementary Information; Figs. S9 – S11 ). However, this increased scatter has a minimal impact on detected trends.